Zinc-finger nickase-mediated insertion of the lysostaphin gene into the beta-casein locus in cloned cows Zinc-finger nickases (ZFNickases) are a type of programmable nuclease that can be engineered from zinc-finger nucleases to induce site-specific single-strand breaks or nicks in genomic DNA, which result in homology-directed repair. Although zinc-finger nuclease-mediated gene disruption has been demonstrated in pigs and cattle, they have not been used to target gene addition into an endogenous gene locus in any large domestic species. Here we show in bovine fetal fibroblasts that targeting ZFNickases to the endogenous β-casein (CSN2) locus stimulates lysostaphin gene addition by homology-directed repair. We find that ZFNickase-treated cells can be successfully used in somatic cell nuclear transfer, resulting in live-born gene-targeted cows. Furthermore, the gene-targeted cows secrete lysostaphin in their milk and in vitro assays demonstrate the milk’s ability to kill Staphylococcus aureus . Our success with this strategy will facilitate new transgenic technologies beneficial to both agriculture and biomedicine. Zinc-finger nickase (ZFN) technology is a powerful tool for genome engineering that enables targeted mutagenesis [1] , [2] , [3] , [4] , [5] , [6] , [7] . ZFNs cleave DNA, producing site-specific double-strand breaks (DSBs) in a genome. DSBs are repaired by non-homologous end joining (NHEJ), which often introduces short insertions or deletions (indels) at the sealed break, or by homology-directed repair (HDR), which faithfully restores the original sequence by copying it from the sister chromatid. These two pathways can be used for site-directed modification of the genome, although NHEJ is the dominant pathway of DSB repair in higher eukaryotic cells and organisms [8] . Currently, ZFNs have been broadly applied to basic research, biotechnology and medicine, but genome engineering with programmable nucleases is limited by the inevitable production of DSBs and the reliance on error-prone NHEJ. Further, these programmable nucleases often induce randomly generated and unwanted indels at highly homologous sites. Furthermore, the nucleases inducing too many off-target DSBs are toxic to cells. Furter, it is difficult to isolate correctly gene-targeted cells [5] , [9] . One potential strategy to overcome this limitation is the targeted introduction into DNA containing a SSB or nick. Like the DSB, a SSB/nick can theoretically stimulate the HDR pathway [10] , [11] , [12] . In contrast to a DSB, it is important that a nick or SSB is not a bona fide substrate for repair by the NHEJ pathway. Thus, a targeted SSB has the potential to restrict repair to the HDR pathway [13] . Lysostaphin, produced naturally by Staphylococcus simulans , has been proposed as a systemic therapy for S. aureus infection [14] . Its efficacy against mastitis caused by S. aureus was demonstrated in a mouse model [15] , [16] . It has been reported that transgenic cattle expressing lysostaphin in their milk could resist S. aureus intramammary infection [17] and that the authentic lysostaphin produced in vitro by a mammalian cell line could result in protein inactivity due to glycosylation [16] . Thus, the coding sequence was modified to generate Gln 125,232 -lysostaphin so that two potential glycosylation sites were removed. This prevented protein glycosylation and restored partial activity [16] . The objective of this study was to perform efficient and reproducible gene targeting in bovine fetal fibroblasts by inserting the exogenous Gln 125,232 -lysostaphin gene into the beta-casein locus so that lysostaphin protein could be produced in the mammary gland of the gene-targeted cow. Assessment of ZFN activity in bovine fetal fibroblasts As the 51-base pair signal peptide sequence of the coding region in the bovine CSN2 gene is located in exon2, an exogenous gene containing splice acceptor sequence addition in intron2 should be successfully targeted to cause the expression of the exogenous gene mimicking endogenous β-casein. Furthermore, the splice acceptor activity was validated in bovine fetal fibroblasts ( Fig. 1 ). Thus, we chose intron 2 of the bovine CSN2 locus for targeting with pairs of ZFNs, using previously described strategy [3] . We designed ZFNs that formed pairs targeting the CSN2 locus and screened them in a budding yeast-based system to rapidly measure their ZFN activity ( Fig. 2a,b ). We then tested the ZFNs for native gene-disruption activity at their target locus in BFFs. The BFFs were transfected with different quantities of plasmids expressing the ZFNs and the frequency of ZFN-mediated disruption at the target site in each pool of cells was determined by the CEL-I nuclease assay ( Fig. 2c ). Both ZFN1/ZFN2 and ZFN3/ZFN4 pairs could cleave, and thereby initiate mutation of, the target locus within the intron2 of CSN2 . However, the ZFN1/ZFN2 pair cleaved the target gene more efficiently than the ZFN3/ZFN4 pair, as demonstrated by the increased incidence of allelic mutations (NHEJ frequency), particularly at higher levels of input ZFNs ( Fig. 2c ). Therefore, we used the ZFN1/ZFN2 pair in subsequent experiments. 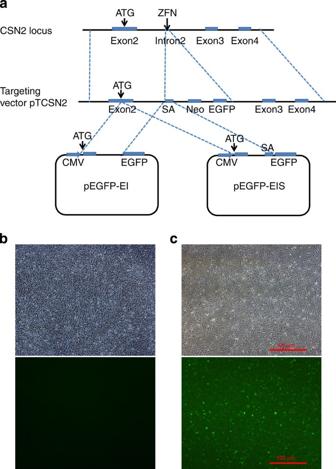Figure 1: Validation of splice acceptor activity in bovine fetal fibroblasts. (a) Schematic overview depicting the verification strategy for the splice acceptor activity. (b) The bovine fetal fibroblasts were transfected by pEGFP-EI. (c) The bovine fetal fibroblasts were transfected by pEGFP-EIS. Scale bars in (b) and (c) represent 100 μm. Figure 1: Validation of splice acceptor activity in bovine fetal fibroblasts. ( a ) Schematic overview depicting the verification strategy for the splice acceptor activity. ( b ) The bovine fetal fibroblasts were transfected by pEGFP-EI. ( c ) The bovine fetal fibroblasts were transfected by pEGFP-EIS. Scale bars in ( b ) and ( c ) represent 100 μm. 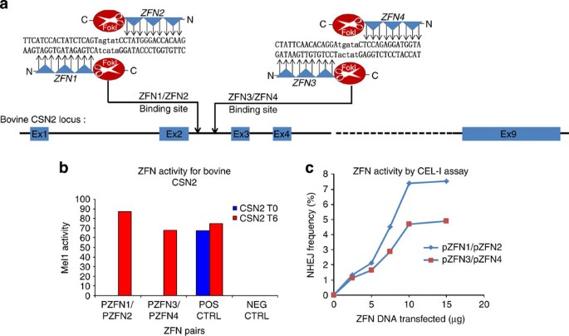Figure 2: Targeting the bovineCSN2locus with ZFNs and ZFNickases. (a) Section of theCSN2gene targeted by ZFNs. Upper part shows cartoons of two pairs of ZFNs binding at specific genomic sites. The DNA sequence of the primary binding site for each ZFN is uppercase. The cut sites cleaved by dimerization of theFokI nuclease domains are lowercase. (b) Validation ofCSN2targeting by ZFNs. The activities of two pairs of ZFNs for theCSN2locus were measured by the yeast MEL-I assay. ZFN cleavage activity was measured before (0 h, blue bars) and after induction of ZFN expression (6 h, red bars). MEL-I levels positively correlate with the ability of ZFNs to create double-strand breaks at the desired target site. ZFNs that showed >50% signal relative to a CCR5 standard ZFN (positive control) at 6 h were regarded as useful for genome editing experiments. (c) Comparison of ZFN activity in bovine fibroblasts. Plasmids encoding each pair of ZFNs (ZFN1/ZFN2 and ZFN3/ZFN4) containing the ELKK FokI variant were delivered to bovine fibroblasts in the amounts shown. The frequency of allelic mutation in each pool of treated cells was determined using the CEL-I assay. The frequency of NHEJ is plotted against ZFN dosage. Full size image Figure 2: Targeting the bovine CSN2 locus with ZFNs and ZFNickases. ( a ) Section of the CSN2 gene targeted by ZFNs. Upper part shows cartoons of two pairs of ZFNs binding at specific genomic sites. The DNA sequence of the primary binding site for each ZFN is uppercase. The cut sites cleaved by dimerization of the Fok I nuclease domains are lowercase. ( b ) Validation of CSN2 targeting by ZFNs. The activities of two pairs of ZFNs for the CSN2 locus were measured by the yeast MEL-I assay. ZFN cleavage activity was measured before (0 h, blue bars) and after induction of ZFN expression (6 h, red bars). MEL-I levels positively correlate with the ability of ZFNs to create double-strand breaks at the desired target site. ZFNs that showed >50% signal relative to a CCR5 standard ZFN (positive control) at 6 h were regarded as useful for genome editing experiments. ( c ) Comparison of ZFN activity in bovine fibroblasts. Plasmids encoding each pair of ZFNs (ZFN1/ZFN2 and ZFN3/ZFN4) containing the ELKK FokI variant were delivered to bovine fibroblasts in the amounts shown. The frequency of allelic mutation in each pool of treated cells was determined using the CEL-I assay. The frequency of NHEJ is plotted against ZFN dosage. Full size image Mutation of the ZFN catalytic domain generates a ZFNickase To generate ZFNs with strand-specific nicking activity, we mutated the Fok I catalytic domain in one of the two ZFNs necessary for dimerization and subsequent DNA cleavage [18] . Specifically, we focused on amino acid D450, which has been shown to result in catalytically inactive Fok I when mutated [19] . To test the activity of ZFNs bearing D450A point mutations, we digested a linear 366-bp PCR fragment of the CSN2 gene containing an off-centre target site for CSN2 -specific ZFNs ( Fig. 3a,b ). The use of in vitro -synthesized, wild-type CSN2 -specific ZFNs (ZFN1 and ZFN2) resulted in efficient double-strand cleavage of the template DNA into two smaller fragments (>70% cleavage efficiency), regardless of whether the products were resolved by polyacrylamide gel electrophoresis (PAGE) under nondenaturing ( Fig. 3c , lane 1) or denaturing ( Fig. 3c , lane 3) conditions. When coupled with the wild-type right-hand ZFN (ZFN2), introduction of the D450A mutation into ZFN1 eliminated double-strand cleavage ( Fig. 3c , lane 2). To confirm strand-specific nicking activity, the same cleavage products were resolved under denaturing conditions to separate the two single-stranded DNA molecules. As expected, the D450A mutation largely eliminated cleavage of one of the two DNA strands, which was observed as the persistence of the full-length, linear single-stranded template ( Fig. 3c , lane 4). Together, these data demonstrate that elimination of cleavage activity in one half of a ZFN pair by the introduction of a D450A mutation results in the generation of a potent, strand-specific ZFNickase. It is consistent with a recent report that described the construction of nickases using Fok I domain variants with an Asp 450 to Ala mutation [20] . 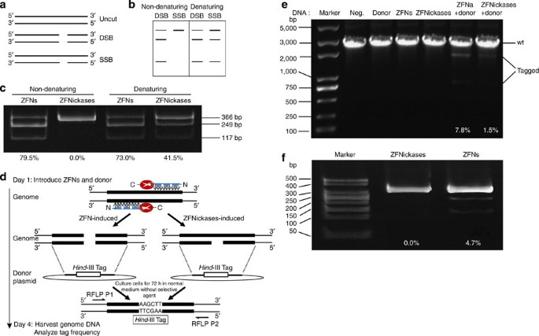Figure 3: ZFNickases-induced SSBs stimulate gene addition in the bovine CSN2 locus. (a) Illustration of the DNA products followingin vitrocleavage with the indicated WT and mutant ZFN combinations and the anticipated cleavage events indicated. (b) Illustration of the expected digestion patterns following strand-specific nicking when resolved under nondenaturing and denaturing conditions. Strand-specificity is revealed because the cleavage site is off-centre. (c)In vitroassessment of double-strand DNA cleavage with the ZFN1/ZFN2 and ZFN1-D450A/ZFN2 variants under nondenaturing conditions and denaturing conditions. Numbers at the bottom of each lane indicate % of cleaved products. (d) Experimental outline and a schematic of the process whereby a ZFN-induced DSB or a ZFNickases-induced SSB is repaired by using an extrachromosomal donor as a template. (e) PCR-based measurements of ZFN-driven tag integration frequency into the CSN2 locus in bovine fibroblasts. Cells were left untransfected (lane 2, ‘neg.’ for negative control) or were transfected with donor plasmids carrying aHindIII-tag flanked by 700-bp homology arms (lane 3) and expression cassettes for ZFNs that induce a DSB or ZFNickases that induce a SSB at intron 2 of CSN2 in the absence (lane 4, 5) and presence (lane 6, 7) of the donor plasmids. Genomic DNA was extracted 72 h later. The percentage ofHindIII -sensitive DNA is indicated below the lane 6 and lane 7. (f) The samples in panel e (lane 6, 7) were also analysed for the presence of indels using the Surveyor nuclease assay. Numbers at the bottom of each lane indicate the percentage of CSN2 alleles containing indels. Figure 3: ZFNickases-induced SSBs stimulate gene addition in the bovine CSN2 locus. ( a ) Illustration of the DNA products following in vitro cleavage with the indicated WT and mutant ZFN combinations and the anticipated cleavage events indicated. ( b ) Illustration of the expected digestion patterns following strand-specific nicking when resolved under nondenaturing and denaturing conditions. Strand-specificity is revealed because the cleavage site is off-centre. ( c ) In vitro assessment of double-strand DNA cleavage with the ZFN1/ZFN2 and ZFN1-D450A/ZFN2 variants under nondenaturing conditions and denaturing conditions. Numbers at the bottom of each lane indicate % of cleaved products. ( d ) Experimental outline and a schematic of the process whereby a ZFN-induced DSB or a ZFNickases-induced SSB is repaired by using an extrachromosomal donor as a template. ( e ) PCR-based measurements of ZFN-driven tag integration frequency into the CSN2 locus in bovine fibroblasts. Cells were left untransfected (lane 2, ‘neg.’ for negative control) or were transfected with donor plasmids carrying a Hin dIII-tag flanked by 700-bp homology arms (lane 3) and expression cassettes for ZFNs that induce a DSB or ZFNickases that induce a SSB at intron 2 of CSN2 in the absence (lane 4, 5) and presence (lane 6, 7) of the donor plasmids. Genomic DNA was extracted 72 h later. The percentage of Hin dIII -sensitive DNA is indicated below the lane 6 and lane 7. ( f ) The samples in panel e (lane 6, 7) were also analysed for the presence of indels using the Surveyor nuclease assay. Numbers at the bottom of each lane indicate the percentage of CSN2 alleles containing indels. Full size image ZFNickase-mediated gene modification at an endogenous locus To investigate whether ZFNickases could promote efficient addition of a small DNA fragment at a predetermined endogenous locus in mammalian cells, we built a donor DNA plasmid engineered to introduce a Hin dIII recognition site tag in-frame with the endogenous locus ( Fig. 3d ). In this construct, a 1,476-bp homology arm isogenic to the CSN2 locus was interrupted with a 6-bp sequence engineered to introduce a Hin dIII recognition site (generating a restriction fragment length polymorphism (RFLP)). Importantly ( Fig. 3d ), the tag was placed precisely at the position of the ZFN-induced break. We introduced this donor plasmid along with an expression plasmid encoding a ZFNickase engineered to introduce a SSB in intron2 of CSN2 into BFFs. Cotransfection of the CSN2 -fragment donor with the ZFN1/ZFN2 pair (DSB-inducing) resulted in transfer of the RFLP to the chromosome at a frequency of 7.8% of the endogenous CSN2 alleles in the absence of positive selection ( Fig. 3e , lane 6). In addition, BFFs cotransfected with the ZFN1-D450A/ZFN2 ZFNickase pair (SSB-inducing) also led to the introduction of the RFLP into the endogenous CSN2 locus at a frequency of 1.5% ( Fig. 3e , lane 7). RFLP addition could not be detected in any samples treated without ZFNs or ZFNickases ( Fig. 3e , lanes 2–5). Analysis of identical ZFNs/ZFNickases-treated BFF pools using the Surveyor Nuclease assay revealed the indels in 4.7% of CSN2 alleles when the DSB-inducing ZFN1/ZFN2 pair was used ( Fig. 3f , lane 3). In contrast, no NHEJ events were detected in samples treated with the ZFN1-D450A/ZFN2 ZFNickase ( Fig. 3f , lane 2). Taken together, these results suggest that a targeted DNA nick at the CSN2 locus can be repaired by HDR (exploiting the RFLP-containing donor DNA fragment), and such nicks do not generate the indels characteristic of the NHEJ repair pathway. ZFNickases promote HDR-mediated site-specific gene addition We constructed the gene-targeting vector, pCSN2-Lys-Neo-EGFP, by inserting the mature portion of the lysostaphin gene with splice acceptor sequence into the Hin dIII site of the CSN2 -fragment donor ( Fig. 4a,b ). We introduced this targeting vector along with expression plasmids encoding ZFNs/ZFNickases engineered to introduce a DSB/SSB in intron 2 of CSN2 into BFFs ( Fig. 4c,d ). Two different early-passage (P2 or P3) primary BFF cell lines were used for transfection: a female cell line, BFF 0911, and a male cell line, BFF1101 ( Table 1 ). Stably transfected cells present in target cell populations were identified following 7–9 days of (600 μg ml −1 ) G418 selection. 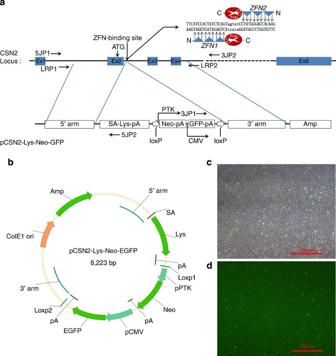Figure 4: Targeting of CSN2 in bovine fibroblasts. (a) Schematic overview depicting the targeting strategy for the CSN2 locus. Blue boxes, exons of CSN2; vertical arrowline, the translational initiation signals (ATG) of the β-casein; bold vertical arrowline, genomic site cut by the respective ZFN pair; level arrow lines, primers used for junction PCR and long-range PCR; The positions and orientations of the loxP sites are indicated as hollow arrows. Shown above is a schematic of the donor plasmid design. Donor plasmid was created corresponding to the cleavage location of the ZFN pairs and carried each roughly 700-bp regions of homology to the CSN2 sequence astride the cleavage site. SA, splice acceptor sequence; Lys, Lysostaphin gene sequence; pA, polyadenylation signals; Neo, the neomycin resistance gene; GFP, the enhanced green fluorescent protein gene; PTK, protein tyrosine kinase promoter; CMV, human cytomegalovirus immediate early promoter; Amp, Ampicillin resistance gene. Inset at upper right is a cartoon of two ZFNs binding at a specific genomic site (uppercase), leading to dimerization of the FokI nuclease domains. (b) Vector maps of gene-targeting vector pCSN2-Lys-Neo-GFP. (c,d) The bovine fibroblasts were transfected by gene-targeting vector pCSN2-Lys-Neo-GFP, c is the bright field view of d. Scale bars represent 100 μm. Figure 4: Targeting of CSN2 in bovine fibroblasts. ( a ) Schematic overview depicting the targeting strategy for the CSN2 locus. Blue boxes, exons of CSN2; vertical arrowline, the translational initiation signals (ATG) of the β-casein; bold vertical arrowline, genomic site cut by the respective ZFN pair; level arrow lines, primers used for junction PCR and long-range PCR; The positions and orientations of the loxP sites are indicated as hollow arrows. Shown above is a schematic of the donor plasmid design. Donor plasmid was created corresponding to the cleavage location of the ZFN pairs and carried each roughly 700-bp regions of homology to the CSN2 sequence astride the cleavage site. SA, splice acceptor sequence; Lys, Lysostaphin gene sequence; pA, polyadenylation signals; Neo, the neomycin resistance gene; GFP, the enhanced green fluorescent protein gene; PTK, protein tyrosine kinase promoter; CMV, human cytomegalovirus immediate early promoter; Amp, Ampicillin resistance gene. Inset at upper right is a cartoon of two ZFNs binding at a specific genomic site (uppercase), leading to dimerization of the FokI nuclease domains. ( b ) Vector maps of gene-targeting vector pCSN2-Lys-Neo-GFP. ( c , d ) The bovine fibroblasts were transfected by gene-targeting vector pCSN2-Lys-Neo-GFP, c is the bright field view of d. Scale bars represent 100 μm. Full size image Table 1 Summary of PCR results of G418-resistant colonies. Full size table Drug-resistant colonies were trypsinized and screened for targeting events by 5′ junction PCR using primers 5JP1 and 5JP2 specific for the CSN2 locus and the Lysostaphin gene to confirm whether stable genetic modification of cells in each of these experimental groups was brought about by targeted or random DNA insertion ( Fig. 4a ). From a total of four transfections in two different cell lines, 1138 G418-resistant colonies were picked, and 131 colonies (11.5%) of them were positive for CSN2 gene targeting in the initial 5′ junction PCR screen (range 4.2–21.5% for the different transfections; Table 1 ). To rule out potential false positives, we used 3′ junction PCR on genomic DNA from 5′ junction PCR-positive colonies using primers 3JP1 and 3JP2 to amplify the right-hand junction between endogenous and exogenous DNA ( Fig. 4a ). Next, we carried out a long-range PCR with both primers (LRP1 and LRP2) located outside the recombination region ( Fig. 4a ). We found that 8.7% (99) of the G418-resistant colonies contained correctly targeted cells ( Table 1 ). A few targeted colonies senesced before they could be prepared for nuclear transfer. The karyotype of each colony was checked; all had chromosome numbers in a range similar to that of freshly isolated BFF cells (≈80% of spreads with 60 chromosomes). Finally, 69 colonies were available for selecting a clonal targeted population with a stable karyotype that could be expanded for nuclear transfer ( Table 1 ). Nuclear transfer to produce gene-targeted cows To rule out random integration of the transgene, we deployed Southern blot analyses of Bgl II-digested genomic DNA extracted from junction PCR and long-range PCR-positive colonies ( Fig. 5 ). Sixteen targeted colonies were used for Southern blot analyses (eight colonies from ZFNickases-induced group and eight colonies from ZFNs-induced). As shown in Fig. 5 , only one clone (lane 8) contained a second, random integration of the transgene. Then, 12 targeted colonies without random integration were prepared for somatic cell nuclear transfer (SCNT). Finally, 5,799 embryos were successfully reconstructed, 1,671 reconstructed embryos were developed to blastocyst stage (the blastocyst formation rates ranged from 25.8 to 31.9%) and no significant difference in cleavage or blastocyst formation rate was observed among the groups. A total of 559 recipients were used for the embryo transfer. The pregnancy rate of recipients receiving ZFNickase-induced colonies was higher than that for recipients receiving ZFNs-induced colonies ( Table 2 ). Ultimately, 19 of 140 pregnancies developed to term (16 derived from the ZFNickase-induced group and 3 from the ZFN-induced group), yielding 14 live gene-targeted calves, with birth weights between 45 and 55 kg. Six of these calves perished soon after birth but eight lived for >1 month ( Table 2 ). All these defects have frequently been described in cloned cattle [21] , [22] , [23] , [24] , [25] , [26] , [27] . We did not expect abnormal phenotypes as a direct result of the gene-targeting addition using ZFNs or ZFNickases because the donor cells for SCNT were strictly selected for single-copy and site-specific integration of the exogenous gene without off-target insertion in their genomes. Furthermore, we used these kinds of cells for SCNT and they yielded eight live-born gene-targeted cows. 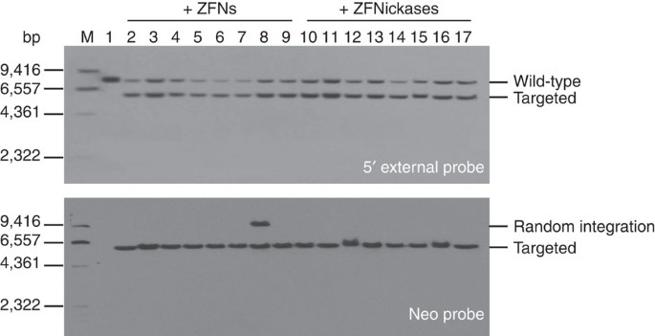Figure 5: Southern blot analysis of the targeted colonies. Lane 1, nontransfected cells were used for negative control. Lanes 2–9, 8 colonies from ZFNs-induced group. Lanes 10–17, 8 colonies from ZFNickases-induced group. Figure 5: Southern blot analysis of the targeted colonies. Lane 1, nontransfected cells were used for negative control. Lanes 2–9, 8 colonies from ZFNs-induced group. Lanes 10–17, 8 colonies from ZFNickases-induced group. Full size image Table 2 Summary of nuclear transfer results from gene-targeted bovine fetal fibroblast cells. Full size table We expected that the calves would be heterozygous for Lys-neo-EGFP cassette knock-in at the CSN2 locus and thus would have one normal copy and one targeted copy of the CSN2 gene ( Fig. 6a ). We used 5′ junction PCR, 3′ junction PCR and long-range PCR to check that the 14 gene-targeted calves, including the 6 that died postnatally, contained a targeted CSN2 locus ( Fig. 6b ). Taq DNA polymerase does not efficiently amplify longer targets (>5 kb), presumably because it lacks 3′→5′ exonuclease activity and cannot correct dNTP misincorporations. The elongation rate from a mismatch is greatly reduced, which decreases the yield of longer products, as indicated by the greater intensity of the long-range PCR band from the nontargeted allele compared with that of the targeted allele. Southern blot analysis was also used to confirm successful targeting. As expected, using Bgl II digestion and a 5′ probe external of the genome homology region, the CSN2 knock-in calves showed two bands: a 7.5-kb band from the endogenous CSN2 allele and a 5.6-kb band characteristic of the insertion ( Fig. 6c , upper). The 5.6-kb band was also detected with a neo probe ( Fig. 6c , lower). 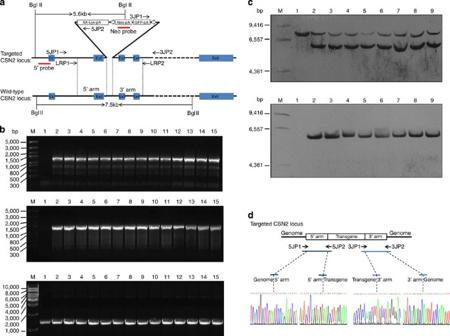Figure 6: Genomic analysis of knock-in cows. (a) Diagram of the bovine CSN2 locus, and the structure of the targeted locus after homologous recombination. The names and positions of the primers used for Junction PCR and long-range PCR are indicated by short arrows. The red bars indicate the probe used for Southern blot analysis. The predicted size of Southern hybridization bands with BglII digestion, for both the endogenous CSN2 locus and the CSN2 targeted locus, is indicated. (b) PCR analysis carried out on chromosomal DNA of nontransgenic cow (lane 1) and of eight gene-targeted calves lived for more than 1 month (lane 2–9) and of six calves perished soon after birth (lane 10–15). 5′junction PCR should yield 1376-bp PCR products using primers 5JP1 and 5JP2 (upper), 3′junction PCR should yield 1419-bp PCR products using primers 3JP1 and 3JP2 (middle), long-range PCR should yield 1.4-kb PCR products (wild-type allele) and 5.4-kb PCR products (targeted allele) using primers LRP1 and LRP2 (lower). The positions and sizes of specific PCR products are indicated at the right. (c) Southern blot analysis of the CSN2 knock-in calves. Lane 1 contains normal cow DNA digested withBglII as a negative control. Lane 2–9 areBglII-digested genomic DNA from eight gene-targeted calves lived for >1 month. Using the external probe 5′ of the genome homology region, theCSN2knock-in calves showed two bands: a 7.5-kb band from the endogenousCSN2allele and a 5.6-kb band characteristic of the insertion (upper). The 5.6-kb band was also detected with a neo probe (lower). (d) Nucleotide sequence analysis of junctions between endogenous and exogenous DNA corresponding to HR events. The 1,376-bp and 1,419-bp PCR products specific for the left- and right- hand junctions are indicated by dark and light blue bars, respectively. Primary nucleotide sequence data corresponding to transition regions between the homology arms of pCSN2-Lys-Neo-GFP and outward host chromosomal DNA and between the homology arms of pCSN2-Lys-Neo-GFP and inward transgene DNA. Figure 6: Genomic analysis of knock-in cows. ( a ) Diagram of the bovine CSN2 locus, and the structure of the targeted locus after homologous recombination. The names and positions of the primers used for Junction PCR and long-range PCR are indicated by short arrows. The red bars indicate the probe used for Southern blot analysis. The predicted size of Southern hybridization bands with BglII digestion, for both the endogenous CSN2 locus and the CSN2 targeted locus, is indicated. ( b ) PCR analysis carried out on chromosomal DNA of nontransgenic cow (lane 1) and of eight gene-targeted calves lived for more than 1 month (lane 2–9) and of six calves perished soon after birth (lane 10–15). 5′junction PCR should yield 1376-bp PCR products using primers 5JP1 and 5JP2 (upper), 3′junction PCR should yield 1419-bp PCR products using primers 3JP1 and 3JP2 (middle), long-range PCR should yield 1.4-kb PCR products (wild-type allele) and 5.4-kb PCR products (targeted allele) using primers LRP1 and LRP2 (lower). The positions and sizes of specific PCR products are indicated at the right. ( c ) Southern blot analysis of the CSN2 knock-in calves. Lane 1 contains normal cow DNA digested with Bgl II as a negative control. Lane 2–9 are Bgl II-digested genomic DNA from eight gene-targeted calves lived for >1 month. Using the external probe 5′ of the genome homology region, the CSN2 knock-in calves showed two bands: a 7.5-kb band from the endogenous CSN2 allele and a 5.6-kb band characteristic of the insertion (upper). The 5.6-kb band was also detected with a neo probe (lower). ( d ) Nucleotide sequence analysis of junctions between endogenous and exogenous DNA corresponding to HR events. The 1,376-bp and 1,419-bp PCR products specific for the left- and right- hand junctions are indicated by dark and light blue bars, respectively. Primary nucleotide sequence data corresponding to transition regions between the homology arms of pCSN2-Lys-Neo-GFP and outward host chromosomal DNA and between the homology arms of pCSN2-Lys-Neo-GFP and inward transgene DNA. Full size image Finally, we tested whether the junctions between CSN2 and the inserted DNA were precise at the nucleotide level. We PCR-amplified the left- and right-hand junctions between the endogenous and exogenous DNA from gene-targeted calves using primer sets 5JP1 plus 5JP2 and 3JP1 plus 3JP2, respectively ( Fig. 6d ). We cloned and sequenced the resulting 1,376-bp and 1,419-bp fragments. There were no point mutations or micro-rearrangements (such as indels) on either side of the two homology arms ( Fig. 6d ). These results, together with those of the PCR ( Fig. 6b ) and Southern blotting ( Fig. 6c ) firmly demonstrate the capacity of ZFNickases with sequence- and strand-specific endonuclease activity to trigger homology-directed insertion of a functional expression unit at a native locus in the bovine genome. Prepubertal gene-targeted calves (GT12120 and GT12128), 4–5 months old and weighing 90–150 kg, were induced to lactate as previously described [28] . The expression of the exogenous lysostaphin gene was expected to mimic that of endogenous β-casein. Indeed, lysostaphin protein was present in milk from two transgenic cows, but not in that from a nontransgenic cow ( Fig. 7a ). Moreover, there was a clear reduction in CSN2 expression in transgenic cows compared with the nontransgenic cow ( Fig. 7b ). We demonstrated the bacteriolytic activity of the milk from the transgenic cows using a lysis assay in which milk samples were incubated on a lawn of S. aureus ( Fig. 7c ). Judging from western blot analysis of milk probed with antibody against recombinant lysostaphin for transgenic animals GT12120 and GT12128 the concentration of lysostaphin in the transgenic milk is ~5 ng μl −1 ( Fig. 7a ). The in vitro biological activity for 50 ng (10 μl transgenic milk) transgenically produced lysostaphin was equivalent to 5 ng of recombinant lysostaphin ( Fig. 7c ), which indicates that the transgenically produced protein is ~10% as active as bacterially derived recombinant lysostaphin. 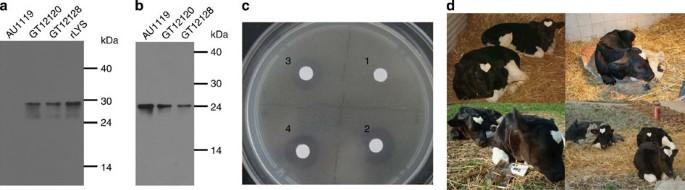Figure 7: Analysis of lysostaphin protein expression in milk of knock-in cows. (a) Western blot analysis of milk probed with antibody against recombinant lysostaphin: 1 μl milk from gene-targeted cows GT12120, GT12128 and nontransgenic cow AU1119. Bacterially derived recombinant lysostaphin in saline (10 ng). (b) Western blot analysis for the expression of β-casein: 1 μl milk from gene-targeted cows GT12120, GT12128 and nontransgenic cow AU1119 were used. (c) Bacterial plate assay for staphylolytic activity. Lytic zones developed on a lawn ofS. aureus12 h after sample application: 10 μl milk from nontransgenic cow (1) and 10 μl (500 ng ml−1) recombinant lysostaphin (2) and 10 μl milk from gene-targeted cows (3, 4). (d) Eight gene-targeted calves lived for more than one month. Figure 7: Analysis of lysostaphin protein expression in milk of knock-in cows. ( a ) Western blot analysis of milk probed with antibody against recombinant lysostaphin: 1 μl milk from gene-targeted cows GT12120, GT12128 and nontransgenic cow AU1119. Bacterially derived recombinant lysostaphin in saline (10 ng). ( b ) Western blot analysis for the expression of β-casein: 1 μl milk from gene-targeted cows GT12120, GT12128 and nontransgenic cow AU1119 were used. ( c ) Bacterial plate assay for staphylolytic activity. Lytic zones developed on a lawn of S. aureus 12 h after sample application: 10 μl milk from nontransgenic cow (1) and 10 μl (500 ng ml −1 ) recombinant lysostaphin (2) and 10 μl milk from gene-targeted cows (3, 4). ( d ) Eight gene-targeted calves lived for more than one month. Full size image Here we demonstrate the feasibility of a ZFNickase-stimulated gene addition at endogenous bovine loci and the successful production of cloned cows by SCNT using ZFNickase-targeted cells. ZFNickase-mediated gene addition is superior to conventional ZFN targeting because of its high efficiency and the absence of significant mutagenesis by the error-prone NHEJ repair pathway [20] , [29] . The application of transgenesis to direct the expression of foreign protein into mouse milk was first reported in 1987 (ref. 30 ). Lactation-specific transgenes have since been incorporated into pigs [31] , sheep [32] , goats [33] and cattle [34] , and they were primarily intended for pharmaceutical interests that were seeking to generate animal bioreactors. The mammary production of antibacterial proteins for enhanced mastitis resistance has been proposed as a prime agricultural application of this technology [15] , [35] . Antibacterial activity has been observed in the milk from transgenic cows that were engineered to produce lysostaphin in milk [17] . However, the technology that was used then was simply the random integration of the transgene that contained lysostaphin and the beta-lactoglobulin regulatory region. In this study, we report a technology that enables the production of precisely engineered transgenic cattle. We have successfully inserted the bacterial lysostaphin gene into the beta-casein gene locus of calves. When these calves were induced to lactate, the milk contained lysostaphin that had antibacterial activity. This represents a step towards the eventual FDA approval of transgenic animals because the transgene can be inserted into a pre-defined locus. The method of development for cell-mediated transgenesis based on SCNT provides an opportunity to shape the genetic make-up of livestock animals in a much more directed approach than traditional animal breeding and selection schemes. Progress in the site-directed modulation of livestock genomes is currently limited by the low efficiency of gene targeting that is imposed by the low frequency of homologous recombination and the limited proliferative capacity of primary somatic cells that are used to produce transgenic animals. Recent new technologies enable targeted editing of genomes in diverse systems. This includes the precise manipulation of gene sequences in their natural chromosomal context and the addition of transgenes to specific genomic loci. This progress has been facilitated by advances in engineering targeted nucleases with programmable, site-specific DNA-binding domains, including zinc-finger proteins and transcription activator-like effectors (TALEs). The enhancement of gene targeting through nuclease-mediated DNA cleavage has been known for over 15 years, but genome editing has not been widely applied to produce livestock species so far [1] , [7] , [36] , [37] , [38] . CRISPR-mediated genome engineering has also have been studied in zebrafish [39] and in human cells [40] , which demonstrated a broad application of this new technology. These studies implied that the CRISPR system can provide the next-next generation of targetable cleavage reagents to produce livestock species. Recently, two independent studies on ZFNickases modified CCR5-specific ZFNs to make ZFNickases and showed that these nickases did not induce significant levels of indels at the target site [13] and that ZFNickases did not induce mutagenic NHEJ at any measurable frequency by using conventional DNA sequencing, deep sequencing and the T7E1 assay [20] . Another study recently demonstrated that a TALEN nickase can effect target gene correction at an endogenous locus [41] . For applications in stem cell research and gene therapy, in which off-target mutations are of concern, precise genome editing with nickases would be preferred. In conclusion, the relatively high percentage of integration of a long DNA fragment into a predetermined locus in the bovine genome demonstrates that ZFNickases are active in BFFs. Just like ZFNs, ZFNickases can be used to produce knock-in cows by SCNT. ZFNickases can be engineered against a broad range of endogenous genes within a few weeks and ZFNickase-driven gene addition and the generation of knock-in cows by cloning can be accomplished within 10 months. ZFNickases, unlike their corresponding nucleases, allowed efficient gene-targeting addition at the target site without or with less inducing unwanted random integration of the transgene ( Table 3 , Fig. 8 ). We propose that programmable nickases are novel tools for precision genome engineering, enabling targeted gene addition in any cells or organisms. Our success with this strategy will facilitate a range of new transgenic technologies beneficial to both agriculture and biomedicine. Table 3 Summary of ZFNs/ZFNickases targeting efficiencies for the bovine CSN2 loci in bovine fetal fibroblast cells. 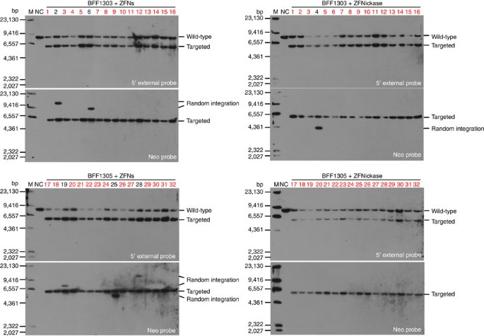Figure 8: Southern blot analysis of BFFs targeted with the indicated ZFN pairs using the corresponding donor plasmid. Genomic DNA was digested withBglII and hybridized with the external 5′ probe or internal neo probe. Correctly targeted clones without additional integrations are indicated in red. Fragment sizes: for 5′ probe and neo probe, wt, 7.5 kb, targeted, 5.6 kb. Full size table Figure 8: Southern blot analysis of BFFs targeted with the indicated ZFN pairs using the corresponding donor plasmid. Genomic DNA was digested with Bgl II and hybridized with the external 5′ probe or internal neo probe. Correctly targeted clones without additional integrations are indicated in red. Fragment sizes: for 5′ probe and neo probe, wt, 7.5 kb, targeted, 5.6 kb. Full size image Construction and validation of ZFNs and ZFNickases ZFNs targeting intron 2 of the bovine CSN2 gene were designed and constructed by Sigma-Aldrich (St Louis, MO, USA, Lot Number: 08181029MN).The design, cloning and validation of the ZFNs was performed by Sigma-Aldrich. ZFN design involved using an archive of pre-validated two-finger and one-finger modules. The target region was scanned for positions where modules exist in the archive. This allowed the fusion of two or three such molecules to generate a five-finger protein that recognizes an 18-bp site on the bottom strand and the fusion of two to three different modules that recognize a 16-bp site on the top strand that lies 5 bp away. The ZFNickases with strand-specific nicking activity were generated by introducing a Fok I domain D450A mutation into the plasmid pZFN1 (which encodes a Left ZFN with Q486E and I499L mutations) using the QuikChange Site-Directed Mutagenesis kit (Stratagene, Carlsbad, CA, USA, Catalogue: 200518) [19] . The residue number of each mutation refers to its position in the full-length Fok I endonuclease. In vitro DNA cleavage assay A 1.4-kb fragment of the CSN2 locus containing the ZFN target site was cloned into the PMD19-T vector (TaKaRa, Dalian, China, TaKaRa Code: D102A), and used as a template for PCR amplification of a 366-bp fragment of CSN2 using primers: 5′-TACACTATTTCCTCATCTTCCCATTC-3′ and 5′-GTTAGTCTGTTGCTTATTGGTTTA-3′. The resulting PCR product was diluted to 1 ng μl −1 in Fok I buffer consisting of 20 mM Tris-HCl, pH 8.5, 150 mM NaCl, 2 mM MgCl 2 , 5% ( v / v ) glycerol, 10 mM ZnCl 2 , 0.5 mg ml −1 BSA and 1 mM DTT. The ZFNs were synthesized in vitro using the TNT T7 Quick Coupled Transcription/Translation System (Promega, Madison, WI, USA, Catalogue: L1170) according to the manufacturer’s recommendations. The appropriate ZFNs and the 366-bp target DNA were mixed in Fok I buffer and incubated at 37 °C for 2 h. The target DNA was then extracted with a phenol/chloroform mixture and either not treated (double-stranded DNA) or treated (single-stranded DNA) with a glyoxal/DMSO solution (1.0 M glyoxal, 10 mM NaH 2 PO 4 /Na 2 HPO 4 , pH 7.0, ≈50% vol/vol DMSO) at 50 °C for 1 h [42] . Double-stranded or single-stranded DNAs were then separated on a 10% PAGE and the gel stained with DuRed nucleic acid gel stain (Fanbo Biochemicals). Cleavage was quantified using ImageJ software. In vivo DNA cleavage assay The frequency of targeted gene mutation in ZFN-treated cells was determined using the CEL-I nuclease assay This assay detects alleles of the target locus that deviate from WT as a result of NHEJ-mediated imperfect repair of ZFN- and ZFNickase-induced DNA breaks. PCR amplification of the targeted region from a pool of ZFN- or ZFNickase-treated cells generates a mixture of WT and mutant amplicons. Melting and reannealing of this mixture results in mismatches forming between heteroduplexes of the WT and mutant alleles using a temperature programme of: 95 °C per 10 min; 95 °C–85 °C (−2 °C s −1 ); 85 °C–25 °C (−0.1 °C s −1 ); 4 °C hold. A DNA ‘bubble’ formed at the site of mismatch is cleaved by the Surveyor enzyme (Transgenomic SURVEYOR Kit, Catalogue No.706025), and the cleavage products are incubated at 42 °C for 20 min and electrophoresed on a 10% TBE polyacrylamide gel (BioRad) and quantified by densitometry. The relative intensity of the cleavage products compared with the parental band is a measure of the level of CLE-I cleavage of the heteroduplex. This reflects the frequency of ZFN- or ZFNickase-mediated cleavage of the endogenous target locus that has subsequently undergone imperfect repair by NHEJ. The sequences of PCR primers used for amplification of the CSN2 target locus were: forward primer, 5′-TACACTATTTCCTCATCTTCCCATTC-3′; reverse primer, 5′-GTTAGTCTGTTGCTTATTGGTTTA-3′. A 366-bp PCR product was generated from WT genomic template. Targeting vector construct The β-casein targeting vector (pCSN2-Lys-Neo-EGFP) was constructed by PCR to include a 1.4-kb homology arm of β-casein (AC_000163).This 1.4-kb homology arm containing the ZFN-binding site (5′-TTCATCCACTATCTCAGTagtatCCTATGGGACCACAAG-3′) was cloned into pMD19-T (TaKaRa). The unique ZFN cut site (5′-agtat-3′) in the center of the ZFN binding site was converted into a Hin dIII site (5′-AAGCTT-3′) using the QuikChange Site-Directed Mutagenesis kit (Stratagene; Catalogue: 200518) and the exogenous lysostaphin gene and marker genes were inserted into the Hin dIII site using standard recombinant DNA techniques. Cell culture and selection Primary fetal bovine fibroblasts were isolated from 35-day-old fetuses. The head and viscera were removed and the remaining tissue was minced with sterile scissors. Explants were cultured on 60-mm culture dishes (Nunclon, Denmark) in ~1 ml of cell culture medium (DMEM/F12 (Gibco, New York, NY, USA), 10% fetal bovine serum (FBS; Hyclone, Logan, UT, USA) and 10 ng ml −1 epidermal growth factor) at 37 °C in 5% CO 2 . In addition, 100 U penicillin and 250 ng amphotericin B (Gibco) were added to inhibit microbial growth. The next day, 3 ml of fresh cell culture medium was added. When the cells from the explants reached 70% confluency, on the third day, they were treated with 0.5 ml TE (0.25% trypsin/0.05% EDTA) and passaged 1:2 or 1:3. Then the cells were trypsinized and frozen in 50% FBS, 40% media and 10% DMSO (Sigma), for long-term storage and future use. When needed, cells were thawed and grown in DMEM/F12 (Gibco) medium supplemented with 15% FBS and incubated at 37 °C in a 5% CO 2 atmosphere. At 70–80% confluency, cells were harvested by trypsinization and 9–10 million cells were resuspended in 2 ml Opti-MEM (Gibco). The cells were placed in a 4 mm gap cuvette with 10 μg of the targeting vector (pCSN2-Lys-Neo-EGFP) and 5 μg of the ZFNs-encoding plasmids or ZFNickases-encoding plasmids, and electroporated at 510 V with three pulses of 1 ms duration using the BTX Electro-cell manipulator ECM2001. Electroporated cells were mixed with fresh cell culture medium and plated on 10 cm plates at 5 × 10 5 cells per plate. Three days later, cells were placed in culture medium containing 600 μg ml −1 G418 (Sigma) for 6 days. Cell clones were then collected for PCR screening. Detection of gene-targeting events by PCR G418-positive cell clones derived from cell population transfected with targeting vector pCSN2-Lys-Neo-GFP and either the ZFN or ZFNickases-encoding plasmids were trypsinized and screened for targeting events by PCR. An aliquot of the trypsinization solution (1/3 of the cells) was plated in culture medium containing serum and expanded (for Southern analysis and cryopreservation), while the remaining cells were pelleted. Cell pellets were resuspended in 50 μl PCR lysis buffer (10 mM Tris-HCl pH 8.5, 50 mM KCl, 1.5 mM MgCl 2 , 0.5% NP-40, 0.5% Tween-20 and 400 μg ml −1 proteinase K). Samples were incubated at 65 °C for 1 h, followed by inactivation of proteinase K at 95 °C for 10 min. Five microlitres of the DNA lysate were then used for PCR. Cellular DNA extracted from parental nontransfected cells served as negative control. Five microliters of the DNA lysate were subjected to PCR with the left-hand CSN2-transgene junctions primers (5’J P1: 5′-TTATGTGGGACAAAGGGGAGA-3′; 5′J P2: 5′-TTCCCGCCTCCATAGTTAGACC-3′), the right-hand CSN2-transgene junctions primers (3’J P1: 5′-CGCCGACCACTACCAGCAGAACAC-3′; 3′J P2: 5′-CAGGCTCCTCCTCTATGGGATTTT-3′), and the long-range PCR primers (LRP1: 5′-TCCCAGAATCTAAGACAT-3′; LRP2: 5′-TTGCCTCTGAATGAACAC-3′). Fifty microliter PCR mixtures containing 0.2 mM of each primer, 80 mM dNTPs, 0.6 U of LA Taq DNA polymerase and LA PCR bufferII (TaKaRa) at 1 × final concentration were placed in a DNA thermal cycler. PCR products representing left- and right-hand CSN2-transgene junctions were cloned into pMD19-T (TaKaRa), and sent to GenScript (Nanjing) Co., Ltd. for sequencing. Western blot analysis Prepubertal female cows 4–5 months old and weighing 90–150 kg were induced to lactate. The cows were given daily intramuscular injections of 17β-Estradiol (0.1 mg kg −1 body weight, Abcam) and progesterone (0.25 mg kg −1 , Sigma) for 7 d. Dexamethasone (20 mg day −1 , Sigma) was administered intramuscularly on days 18–21. Milk was collected by hand in an aseptic manner for the next 5 d. All samples were centrifuged at 4,000 g for 10 min at 4 °C. One microliter of milk from gene-targeted cows, GT12120 and GT12128, and nontransgenic cow, AU1119, was used for western blot analysis. The primary antibody(1:2,000) used to detect lysostaphin was from AIC BIOTECH (Rockville, MD, USA, Catalogue No.PAb102) and the antibody for β-casein was from Uscn Life Science Inc. (Catalogue No. A98332Bo01). Nuclear transfer All experiments were approved by Care and Use of Animals Center, Northwest A&F University. This study was carried out in strict accordance with the Guidelines for the Care and Use of Animals of Northwest A&F University. Ovaries were collected from the local abattoir and transported to the laboratory within 4–6 h in sterile saline at 20 °C. Cumulus–oocyte complexes (COCs) were aspirated from 4 to 8 mm antral follicles. Only COCs with compact cumulus and evenly granulated cytoplasm were collected and incubated in bicarbonate-buffered tissue culture medium 199 (TCM-199; Gibco, BRL, Grand Island, NY, USA) supplemented with 10% ( v / v ) FCS, 0.075 IU ml −1 human menopausal gonadotropin (HMG), 1 μg ml −1 17-estradiol and 20 ng ml −1 epidermal growth factor (EGF) for 20–22 h at 38.5 °C in 5% CO 2 in air. Cumulus cells were stripped from COCs in PBS containing 0.2% bovine testicular hyaluronidase and incubated in PBS containing 5 μg ml −1 cytochalasin B (CB) and Hoechst 33,342 10 μg ml −1 for 10 min prior to enucleation. Matured oocytes were enucleated by aspirating the PB and a small amount of surrounding cytoplasm in microdrops of PBS supplemented with 5 μg ml −1 cytochalasin B (CB) and 10% FBS. The aspirated cytoplasm was examined under ultraviolet radiation to confirm that the nuclear material had been removed. Nuclear donor cells were induced in G0/G1 phase of cell cycle by serum deprivation prior to use for SCNT. The disaggregated donor cell was injected into the pre-vitelline space of enucleated oocytes. The oocyte–cell couplet was sandwiched with a pair of platinum electrodes connected to the micromanipulator in microdrop of Zimmermann’s fusion medium. A double electrical pulse of 35 V for 10 μs was applied for oocyte–cell fusion. Successfully reconstructed embryos were kept in mSOFaa for 1 h. Reconstructed embryos were activated in 5 μM ionomycin for 4 min, followed by exposure to 1.9 mM dimethylaminopyridine in SOFaa medium for 4 h. Embryos were then cultured in SOFaa medium supplemented with 8 mg ml −1 BSA in a humidified atmosphere of 5% CO 2 in air at 38.5 °C. Fresh day 7 blastocysts were nonsurgically transferred (two embryos per recipient) to the uterine horn ipsilateral to the corpus luteum in Red Angus recipients on the seventh day of standing oestrus. Pregnancy was detected by rectal palpation/ ultrasonography at 90 days of gestation. Southern blot analysis of cow tissues Calf ear biopsies were lysed overnight at 60 °C in a shaking incubator with ~1 ml lysis solution (50 mM Tris-HCl, pH 8.0, 0.15 M NaCl, 10 mM EDTA, 1% SDS, 25% sodium perchlorate, 1% 2-mercaptoethanol and 200 μg ml −1 proteinase K) per 150 mg tissue. DNA was subjected to phenol/chloroform extraction and precipitated with isopropyl alcohol. Resolubilized DNA was treated with RNase A (1 mg ml −1 ) and RNase T1 (1,000 U μl −1 ) at 37 °C for 1 h, then with proteinase K (20 mg ml −1 ) at 55 °C for 1 h. DNA was then extracted with phenol/chloroform, precipitated with ethanol and resuspended in TE buffer. About 10 μg DNA was digested with Bgl II and separated on a 1% agarose gel. Following electrophoresis, DNA was transferred to a nylon membrane and probed a 3′-end digoxigenin-labeled probe. Bands were detected using a chemiluminescent substrate system. Detection of lysostaphin bioactivity Lysostaphin bioactivity was detected in drops (10 μl) of standards or samples that were spotted onto culture plates that had just been streaked with a culture of S. aureus (ATCC 25923). Following overnight incubation (37 °C), bioactivity was observed as lytic zones in the bacterial lawn. Milk samples used in this test were first pasteurized by heating to 63 °C for 30 min. How to cite this article: Liu, X. et al . Zinc-finger nickase-mediated insertion of the lysostaphin gene into the beta-casein locus in cloned cows. Nat. Commun. 4:2565 doi: 10.1038/ncomms3565 (2013).